Two linked pairs ofArabidopsis TNLresistance genes independently confer recognition of bacterial effector AvrRps4 Plant immunity requires recognition of pathogen effectors by intracellular NB-LRR immune receptors encoded by Resistance ( R ) genes. Most R proteins recognize a specific effector, but some function in pairs that recognize multiple effectors. Arabidopsis thaliana TIR-NB-LRR proteins RRS1-R and RPS4 together recognize two bacterial effectors, AvrRps4 from Pseudomonas syringae and PopP2 from Ralstonia solanacearum . However, AvrRps4, but not PopP2, is recognized in rrs1/rps4 mutants. We reveal an R gene pair that resembles and is linked to RRS1 / RPS4 , designated as RRS1B / RPS4B , which confers recognition of AvrRps4 but not PopP2. Like RRS1/RPS4, RRS1B/RPS4B proteins associate and activate defence genes upon AvrRps4 recognition. Inappropriate combinations (RRS1/RPS4B or RRS1B/RPS4) are non-functional and this specificity is not TIR domain dependent. Distinct putative orthologues of both pairs are maintained in the genomes of Arabidopsis thaliana relatives and are likely derived from a common ancestor pair. Our results provide novel insights into paired R gene function and evolution. Plant immunity is activated upon direct or indirect perception of pathogen molecules. Cell surface receptors perceive relatively invariant pathogen molecules such as flagellin or chitin, and intracellular receptors perceive the presence or action of pathogen effectors [1] . The intracellular immune receptors are called resistance (R) proteins and encoded by R genes. Effector recognition by R proteins leads to effector-triggered immunity, which often culminates in programmed cell death, also known as the hypersensitive response (HR) [2] . However, disease resistance can be achieved without HR [3] . Most plant R genes encode nucleotide-binding, leucine-rich repeat (NB-LRR) proteins that structurally and functionally resemble mammalian nucleotide-oligomerization domain-like (NOD-like) receptors [4] . NB-LRR proteins are modular and presumed to undergo intra- and inter-molecular reconfiguration upon effector recognition, activating defence [5] . However, mechanisms of recognition, activation and downstream signalling are poorly understood. R proteins of the TIR-NB-LRR (TNL) subclass carry a Toll/Interleukin-1 receptor/Resistance (TIR) protein domain at their N-termini, with homology to cytoplasmic domains of mammalian and Drosophila transmembrane immune receptors [6] , [7] . Examples include the tobacco N gene for virus resistance [8] , flax L and M genes for flax rust resistance [9] , several Arabidopsis RPP genes for downy mildew resistance [10] , Arabidopsis RPS4 (originally defined as conferring recognition of Pseudomonas syringae pathovar pisi effector AvrRps4) [11] and Arabidopsis RRS1-R that confers resistance to Ralstonia solanacearum via recognition of effector PopP2 (refs 12 , 13 ). The RRS1 - R allele in accession Nd-1 confers PopP2 recognition, whereas the Col-0 RRS1 - S allele does not. RRS1-R (from Ws-2) and RRS1 - S (from Col-0) are required for AvrRps4 recognition by RPS4, and reciprocally RPS4 is required for PopP2 recognition by RRS1-R in Ws-2 (refs 14 , 15 ). RRS1 and RPS4 are adjacent, divergently transcribed and function cooperatively for AvrRps4 and PopP2 recognition, and for resistance to the fungus Colletotrichum higginsianum [14] , [15] . NB-LRRs can require other NB-LRRs for function [16] . For example, RPP2A and RPP2B , two adjacent TNLs in Col-0, are both required for resistance to Hpa race Cala2 (ref. 17 ). Rice RGA4 and RGA5 form a NB-LRR pair for recognition of Avr-Pia and Avr1-CO39, two effectors from the fungal pathogen Magnaporthe oryzae [18] . Tobacco N requires the ‘ N -required gene’ NRG1 (ref. 19 ), and multiple genes of the ADR1 class are required for function of RPS2 , RPP4 and RPP2 (ref. 20 ). In Col-0, mutations in RRS1 or RPS4 do not result in complete loss of resistance to P. syringae pv tomato ( Pst ) strain DC3000 carrying AvrRps4 (refs 14 , 15 , 21 ). Similarly, Ws-2 rrs1-1 and rps4-21 mutants show an HR when infiltrated with Pseudomonas fluorescens ( Pf ) Pf0-1 (a non-pathogenic Pseudomonas strain that carries a type III secretion system) secreting AvrRps4 (refs 22 , 23 ). These data suggest that A. thaliana Ws-2 and Col-0 carry a RRS1- and RPS4 -Independent AvrRps4 Recognition ( RRIR ) locus. To dissect AvrRps4-triggered immunity, we positionally cloned the RRIR locus. We found another pair of R genes, At5g45050 and At5g45060 , highly similar to RRS1 / RPS4 , which confers RRIR, and named the locus as RRS1B/RPS4B . We show using Agrobacterium -mediated transient assays in Nicotiana tabacum that co-expression of RRS1B and RPS4B confers recognition of AvrRps4 but not PopP2. The RRS1B and RPS4B proteins associate with each other, as previously reported for RRS1 and RPS4 (ref. 24 ). Non-authentic R protein associations can also occur between RRS1B and RPS4, and RRS1 and RPS4B, but do not enable effector recognition, suggesting that these R proteins must pair with their appropriate respective partner for function. Although RRS1B/RPS4B does not recognize PopP2, PopP2 still associates in planta with RRS1B. TIR domain exchanges between RRS1 and RRS1B, or between RPS4 and RPS4B, do not compromise function. A chimera in which the C-terminal 3 exons of RRS1-R are exchanged for those of RRS1B confers effector-independent HR in combination with RPS4, but not with RPS4B, suggesting integrity of this region is important to prevent defence signalling before effector perception. We finally compare RRS1 / RPS4 -like gene pairs in several Brassicaceae . These data contribute to understanding TNL-mediated immunity in plants and provide new insights into paired plant immune receptor function and evolution. At5g45050 and At5g45060 co-segregate with the RRIR locus In Ws-2, the RRIR results in HR as well as disease resistance [23] . This is not due to AvrRps4 recognition by RRS1 or RPS4 alone as Pf Pf0-1 (AvrRps4) triggers HR not only in Ws-2 rrs1-1 and rps4-21 single but also in Ws-2 rrs1-1 / rps4-21 double mutants ( Fig. 1 ). No HR was observed in the Ws-2 eds1-1 mutant, suggesting that RRIR is mediated by a TNL R protein ( Fig. 1 ) [25] , [26] . Interestingly, Pf Pf0-1 (PopP2) does not trigger HR in rrs1 - 1 or rps4 - 21 , indicating that the RRIR is specific to AvrRps4 (ref. 23 ). In Col-0, infiltration with either Pst DC3000 or Pf Pf0 1 producing AvrRps4 does not trigger HR, but disease resistance to Pst DC3000 (AvrRps4) is observed ( Figs 1 and 2d ) [3] , [23] . Arabidopsis accession RLD is susceptible to Pst DC3000 (AvrRps4; Supplementary Fig. 1 ) and was crossed with Ws-2 to map RPS4 (ref. 11 ). In addition, RLD does not show HR to Pf Pf0-1 (AvrRps4; Fig. 1 ) [23] indicating absence of RRIR but HR can be observed after Pf Pf0-1 (HopA1) infiltration [27] . To positionally clone the RRIR locus, we analysed a population generated from a cross between Ws-2 rps4-21 and RLD ( Fig. 1 ), segregating for HR to Pf Pf0-1 (AvrRps4). This enabled us to narrow down a region on chromosome 5 close to RRS1/RPS4 containing four TNL-encoding genes ( Fig. 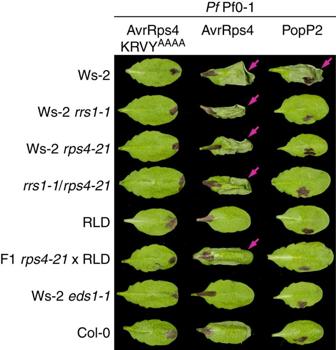Figure 1: AvrRps4 but not PopP2 is recognized in the absence ofRRS1andRPS4. Hypersensitive response (HR) assay in differentArabidopsislines using leaf infiltration withPseudomonas fluorescens(Pf) Pf0-1 secreting AvrRps4 KRVYAAAA, AvrRps4 or PopP2. Pictures were taken 24 h post infiltration (h.p.i.). Magenta arrows indicate leaves showing HR. This experiment was repeated at least three times with similar results. 2a and Supplementary Table 1 ). Among them, At5g45050 and At5g45060 form a pair highly identical to RRS1 / RPS4 ( Fig. 2b ) and were therefore strong candidates for the RRIR locus. Figure 1: AvrRps4 but not PopP2 is recognized in the absence of RRS1 and RPS4 . Hypersensitive response (HR) assay in different Arabidopsis lines using leaf infiltration with Pseudomonas fluorescens ( Pf ) Pf0-1 secreting AvrRps4 KRVY AAAA , AvrRps4 or PopP2. Pictures were taken 24 h post infiltration (h.p.i.). Magenta arrows indicate leaves showing HR. This experiment was repeated at least three times with similar results. 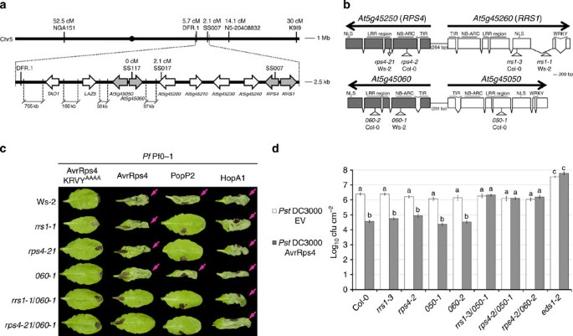Figure 2:At5g45050andAt5g45060conferRRS1/RPS4-independent AvrRps4 recognition (RRIR). (a) Diagram showing the candidateRRIRlocus (grey arrows) onArabidopsischromosome 5. Genetic molecular markers used are shown in uppercase letters with corresponding genetic distance (cM) to theRRIRlocus (based on 48 F2 plants showing no HR to AvrRps4). Arrows represent TNL-encoding genes. Orientation of arrows indicates reading frame direction. The physical distance on the map is indicated in kb or Mb. (b) Schematic representation ofRRS1/RPS4andAt5g45050/At5g45060gene pairs. Positions of the T-DNA insertion for mutant lines used in this study are indicated by white triangles.At5g45050andAt5g45060are abbreviated as050and060, respectively. The mutantsrps4-21(that carries a 5-bp deletion),rrs1-1andrps4-2were reported previously14,15,31. Exons are depicted as boxes, and the different domains are highlighted on the top (APAF1, R proteins and CED4; LRR, leucine-rich repeat; NB-ARC, nucleotide binding, NLS, nuclear localization signal; TIR, Toll/interleukin-1 receptor/R protein; WRKY, WRKY DNA-binding domain). Black arrows indicate the reading frame direction. (c) HR assay in Ws-2 and Ws-2 single and double mutants using leaf infiltration withPfPf0-1 secreting AvrRps4 KRVYAAAA, AvrRps4, PopP2 or HopA1. Pictures were taken 24 h.p.i. Magenta arrows indicate leaves showing HR. (d) Bacterial growth ofPstDC3000 carrying empty vector (EV) or secreting AvrRps4 in Col-0 WT, single and double mutants. Bacterial growth was measured 3 days post infiltration (d.p.i.). Means±standard error (s.e.) of four replicates per sample are given. Samples with different letters are statistically different at the 5% confidence level based on Tukey’s test. These experiments were repeated at least three times with similar results. Full size image Figure 2: At5g45050 and At5g45060 confer RRS1 / RPS4 -independent AvrRps4 recognition (RRIR). ( a ) Diagram showing the candidate RRIR locus (grey arrows) on Arabidopsis chromosome 5. Genetic molecular markers used are shown in uppercase letters with corresponding genetic distance (cM) to the RRIR locus (based on 48 F2 plants showing no HR to AvrRps4). Arrows represent TNL-encoding genes. Orientation of arrows indicates reading frame direction. The physical distance on the map is indicated in kb or Mb. ( b ) Schematic representation of RRS1 / RPS4 and At5g45050/At5g45060 gene pairs. Positions of the T-DNA insertion for mutant lines used in this study are indicated by white triangles. At5g45050 and At5g45060 are abbreviated as 050 and 060 , respectively. The mutants rps4-21 (that carries a 5-bp deletion), rrs1-1 and rps4-2 were reported previously [14] , [15] , [31] . Exons are depicted as boxes, and the different domains are highlighted on the top (APAF1, R proteins and CED4; LRR, leucine-rich repeat; NB-ARC, nucleotide binding, NLS, nuclear localization signal; TIR, Toll/interleukin-1 receptor/R protein; WRKY, WRKY DNA-binding domain). Black arrows indicate the reading frame direction. ( c ) HR assay in Ws-2 and Ws-2 single and double mutants using leaf infiltration with Pf Pf0-1 secreting AvrRps4 KRVY AAAA , AvrRps4, PopP2 or HopA1. Pictures were taken 24 h.p.i. Magenta arrows indicate leaves showing HR. ( d ) Bacterial growth of Pst DC3000 carrying empty vector (EV) or secreting AvrRps4 in Col-0 WT, single and double mutants. Bacterial growth was measured 3 days post infiltration (d.p.i.). Means±standard error (s.e.) of four replicates per sample are given. Samples with different letters are statistically different at the 5% confidence level based on Tukey’s test. These experiments were repeated at least three times with similar results. Full size image At5g45050 and At5g45060 are both required for RRIR To investigate whether the At5g45050/At5g45060 gene pair is the RRIR locus, we tested T-DNA insertion mutants At5g45050-1 ( 050-1 ) in Col-0, At5g45060-1 ( 060-1 ) in Ws-2 and At5g45060-2 ( 060-2 ) in Col-0 ( Fig. 2b and Supplementary Table 2 ), for loss of AvrRps4 recognition. These were crossed to rrs1 or rps4 mutants ( rrs1-1 in Ws-2; rrs1-3 in Col-0; rps4-21 in Ws-2; rps4-2 in Col-0) in order to recover the following double mutants after PCR screening F2 and F3 progenies: Ws-2 rps4-21 / 060-1 , Ws-2 rrs1-1 / 060-1 , Col-0 rrs1-3 / 050-1 , Col-0 rps4-2 / 050-1 and Col-0 rps4-2 / 060-2 . 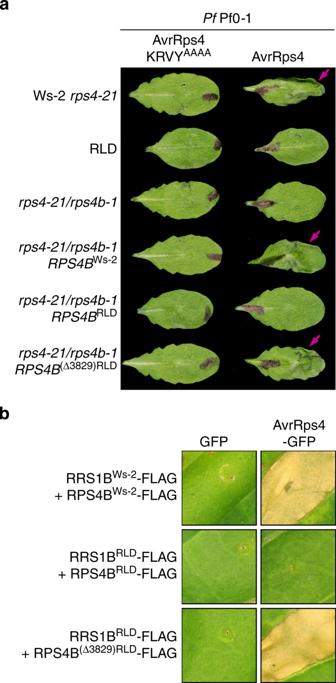Figure 3:RPS4BRLDcarries a mutation responsible for loss of AvrRps4 recognition. (a) HR assay using leaf infiltration withPfPf0-1 secreting AvrRps4 KRVYAAAAor AvrRps4 in Ws-2rps4-21, RLD, Ws-2rps4-21/rps4b-1and stable transgenic lines of Ws-2rps4-21/rps4b-1-expressingRPS4BWs-2,RPS4BRLDorRPS4B(Δ3829)RLD(under native promoter and terminator).RPS4BWs-2andRPS4BRLDwere cloned from accession Ws-2 and RLD, respectively.RPS4B(Δ3829)RLDcorresponds toRPS4BRLDwith the WT inserted nucleotide at position 3,829 bp removed, restoring similar coding sequence to Ws-2. Pictures were taken 24 h.p.i. Magenta arrows indicate leaves showing HR. (b) HR assay inN. tabacumleaves using transientA. tumefacienstransformation. Each leaf section was co-infiltrated to express a combination of differentRgenes (shown on the left) together withGFPoravrRps4-GFP.RRS1,RPS4,RRS1BandRPS4Bwere cloned from Ws-2 or RLD gDNA. Cell death pictures were taken 5 d.p.i. These experiments were repeated at least three times with similar results. Using reverse transcription–PCR (RT–PCR), we confirmed the presence of RPS4 , RRS1 , At5g45060 and At5g45050 transcripts in Ws-2, Col-0, RLD and eds1 mutants; we also confirmed the absence of corresponding transcripts in each single and double T-DNA insertion mutants ( Supplementary Figs 2 and 3 and Supplementary Table 3 ). In rps4-21 , which carries a 5-bp deletion in RPS4 , the transcript was still detected [15] . We then tested AvrRps4 recognition in these single and double mutants. As expected, Ws-2 060-1 mutant showed similar HR to Ws-2 after Pf Pf0-1 (AvrRps4) infiltration, and retained PopP2 recognition and HR due to the presence of RRS1 / RPS4 ( Fig. 2c ). The Ws-2 rrs1-1 and rps4-21 mutants, on the other hand, showed the loss of HR to PopP2, but maintained HR to AvrRps4 ( Fig. 2c ). This residual AvrRps4 recognition and HR was completely abolished in Ws-2 rrs1-1 / 060-1 or rps4-21 / 060-1 double mutants ( Fig. 2c ), suggesting that At5g45060 is required for the RRIR in Ws-2. In addition, rrs1-1 / 060-1 and rps4-21 / 060-1 double mutants showed HR to HopA1 (recognized by the TNL RPS6) [28] , suggesting that HR signalling is still effective in these double mutants. None of the mutants or accessions showed HR to Pf Pf0-1 carrying a mutated AvrRps4 (AvrRps4 KRVY AAAA ), confirming all HR phenotypes resulted from specific effector recognition ( Fig. 2c ) [29] . To test whether loss of HR to AvrRps4 correlates with loss of disease resistance, we assessed the growth of Pst DC3000 (AvrRps4) compared with Pst DC3000 (EV) in wild-type (WT) and Arabidopsis mutants 3 days post infiltration (d.p.i.). AvrRps4 is recognized in Col-0, restricting Pst DC3000 (AvrRps4) growth compared with Pst DC3000 (EV), whereas in Col-0 eds1-2 , Pst DC3000 (AvrRps4) grew as much as Pst DC3000 (EV) ( Fig. 2d ). In Col-0 050-1 and Col-0 060-2 , with the presence of functional RRS1/RPS4 , Pst DC3000 (AvrRps4) growth was restricted compared with Pst DC3000 (EV) ( Fig. 2d ). Similarly, restricted growth of Pst DC3000 (AvrRps4) was observed in Col-0 rrs1-3 and Col-0 rps4-2 due to RRIR ( Fig. 2d ). However, Col-0 rrs1-3 / 050-1 , rps4-2 / 050-1 and rps4-2 / 060-2 double mutants supported as much Pst DC3000 (AvrRps4) growth as Pst DC3000 (EV), indicating the complete loss of AvrRps4 recognition ( Fig. 2d ). Similar results were shown in Ws-2: Pst DC3000 (AvrRps4) grew as well as Pst DC3000 (EV) in Ws-2 rrs1-1 / 060-1 and rps4-21 / 060-1 mutants ( Supplementary Fig. 1 ). This result correlates with the absence of Pf Pf0-1 (AvrRps4)-triggered HR in Ws-2 rrs1-1 / 060-1 and rps4-21 / 060-1 ( Fig. 2c ). Collectively, these data indicate that both At5g45050 and At5g45060 are required for the RRIR in Arabidopsis Ws-2 and Col-0. Because of their strong homology to RRS1 and RPS4 ( Fig. 2b ), At5g45050 and At5g45060 were designated as RRS1B and RPS4B , respectively. Surprisingly, neither rrs1 nor rps4 mutants showed a significant increase in Pst DC3000 (AvrRps4) growth compared with WT Col-0 or Ws-2 ( Fig. 2d and Supplementary Fig. 1 ), in contrast to previous reports [15] , [21] , [29] , most likely due to different growth conditions. RPS4B RLD premature stop codon causes its loss of function The Arabidopsis accession RLD is unable to recognize AvrRps4 and carries a non-functional RPS4 RLD allele ( Fig. 1 and Supplementary Fig. 1 ) [11] , [30] . We compared RRS1B and RPS4B sequences in RLD and Ws-2 to identify polymorphisms that might account for the loss of function. Compared to RRS1B Ws-2 , two non-synonymous substitutions (S586G and I961V) and a deletion of E362 were identified in RRS1B RLD ( Supplementary Fig. 4 ). RPS4B RLD has three non-synonymous substitutions (N264D, C277F and N1053D) and a nucleotide insertion at 3,829 bp, which causes a frame shift and an early stop codon ( Supplementary Fig. 5 ). As a result, RPS4B RLD is missing the C-terminal 63 amino acids (a.a.), including the predicted RPS4B Ws-2 nuclear localization signal (NLS). The integrity of RPS4 NLS was reported to be essential for its immune function [31] . Hence, we speculated that the truncation in RPS4B RLD (causing the loss of NLS) rather than the limited polymorphisms in RRS1B RLD could explain the lack of RRIR in RLD. To test the functionality of RPS4B RLD in Arabidopsis , we transformed Ws-2 rps4-21/rps4b-1 with either RPS4B RLD or RPS4B Ws-2 . As expected, stable transgenic lines of Ws-2 rps4-21/rps4b-1 -expressing RPS4B RLD did not show HR to Pf Pf0-1 (AvrRps4), whereas rps4-21/rps4b-1 -expressing RPS4B Ws-2 did ( Fig. 3a ). This result confirms that RPS4B Ws-2 is able to complement RRIR in Ws-2 rps4-21/rps4b-1 , whereas RPS4B RLD is non-functional. We then restored the full-length RPS4B RLD protein by removing the adenine insertion at position 3829 in RPS4B RLD genomic DNA (gDNA) sequence, and generated RPS4B (Δ3829)RLD that is almost identical to RPS4B Ws-2 . Ws-2 rps4-21/rps4b-1 stably expressing RPS4B (Δ3829)RLD showed HR to Pf Pf0-1 (AvrRps4) at 24 h post infiltration (h.p.i. ; Fig. 3a ), suggesting the C-terminal 63 a.a. present in RPS4B Ws-2 but absent in RPS4B RLD are required for function. Figure 3: RPS4B RLD carries a mutation responsible for loss of AvrRps4 recognition. ( a ) HR assay using leaf infiltration with Pf Pf0-1 secreting AvrRps4 KRVY AAAA or AvrRps4 in Ws-2 rps4-21 , RLD, Ws-2 rps4-21 / rps4b-1 and stable transgenic lines of Ws-2 rps4-21 / rps4b-1- expressing RPS4B Ws-2 , RPS4B RLD or RPS4B (Δ3829)RLD (under native promoter and terminator). RPS4B Ws-2 and RPS4B RLD were cloned from accession Ws-2 and RLD, respectively. RPS4B (Δ3829)RLD corresponds to RPS4B RLD with the WT inserted nucleotide at position 3,829 bp removed, restoring similar coding sequence to Ws-2. Pictures were taken 24 h.p.i. Magenta arrows indicate leaves showing HR. ( b ) HR assay in N. tabacum leaves using transient A. tumefaciens transformation. Each leaf section was co-infiltrated to express a combination of different R genes (shown on the left) together with GFP or avrRps4 - GFP . RRS1 , RPS4 , RRS1B and RPS4B were cloned from Ws-2 or RLD gDNA. Cell death pictures were taken 5 d.p.i. These experiments were repeated at least three times with similar results. Full size image Co-expression of avrRps4 or popP2 , together with RRS1 and RPS4 , by agro-infiltration in N. tabacum leaves results in HR [24] . Using a similar method, we were able to show AvrRps4 recognition by RRS1B/RPS4B in N. tabacum . Co-expression of avrRps4 , but not GFP , together with RRS1B Ws-2 and RPS4B Ws-2 triggered HR at 5 d.p.i. ( Fig. 3b ). We then tested AvrRps4 recognition by RRS1B RLD , RPS4B RLD and RPS4B (Δ3829)RLD using this assay. Consistent with phenotypes observed in Arabidopsis RLD and Ws-2 rps4-21 / rps4b-1 complemented lines, co-expression of RPS4B RLD with either RRS1B RLD or RRS1B Ws-2 in N. tabacum did not show HR to AvrRps4 ( Fig. 3b and Supplementary Fig. 6 ). On the other hand, an AvrRps4-triggered HR was observed when RRS1 B RLD was co-expressed with either RPS4B (Δ3829)RLD or RPS4B Ws-2 ( Fig. 3b and Supplementary Fig. 6 ). The stability of each fusion protein used in the transient assay was verified by western blot analysis ( Supplementary Fig. 7 ). These data suggest that RRS1B RLD is functional and that the insertion causing the premature stop codon in RPS4B RLD is responsible for non-functionality and loss of RRIR in the RLD accession. AvrRps4-induced defence genes require either RPS4 or RPS4B Given two paired R genes that provide resistance to one effector, we investigated the quantitative contributions of RRS1B / RPS4B to AvrRps4-triggered immunity compared with RRS1 / RPS4 by measuring defence gene induction using quantitative RT–PCR. Based on previous studies, we selected defence marker genes ( SARD1 , SID2 , PAD4 and EDS5 ) that are specifically regulated by AvrRps4 and PopP2 in a RRS1 / RPS4 -dependent manner at early stages of immunity [27] . Genotypes Ws-2, Ws-2 rps4-21 , Ws-2 rps4b-1 and rps4-21/rps4b-1 were infiltrated with either H 2 O, Pf Pf0-1-carrying AvrRps4 or AvrRps4 KRVY AAAA mutant. Six hours post infiltration, the fold change of all selected defence marker genes compared with H 2 O treatment was consistently more induced in Ws-2, rps4-21 or rps4b-1 after infiltration with Pf Pf0-1 (AvrRps4) than with Pf Pf0-1 (AvrRps4 KRVY AAAA ; Fig. 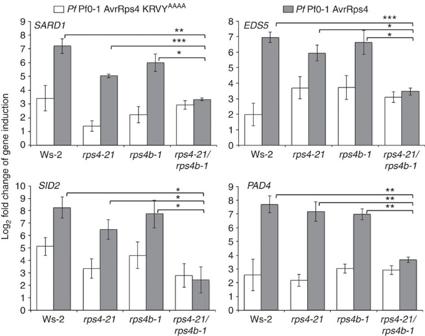Figure 4: Loss ofRPS4andRPS4Bcompletely abolishes AvrRps4-triggered defence gene induction in Ws-2. Quantitative RT–PCR showing fold change ofSARD1,SID2,EDS5andPAD4gene expression. Transcript levels were estimated in leaves of 5-week-old Ws-2, Ws-2rps4-21andrps4b-1single and Ws-2rps4-21/rps4b-1double mutants infiltrated with either H2O,PfPf0-1 secreting AvrRps4 KRVYAAAAor AvrRps4. RNA was extracted from samples taken at 6 h.p.i. for cDNA synthesis. Results of quantitative RT–PCR for selected defence marker genes were first normalized toEF1α, then calculated as log2-scaled fold change compared with H2O treatment. Means±s.e. of three biological replicates per sample are given. Data from individual experiments are shown inSupplementary Fig. 7. Differences that are statistically significant are indicated (Student’st-test *P≤0.05, **P≤0.01, ***P≤0.001). 4 and Supplementary Table 4 ). Assuming that each pair functions independently, this indicates that RRS1B/RPS4B (in rps4-21 ) and RRS1/RPS4 (in rps4b-1 ) were able to activate a similar set of defence genes upon AvrRps4 recognition, and are therefore likely to share downstream signalling mechanisms. In the single knockout mutants tested, there was no consistent pattern of quantitative differences between RRS1/RPS4- and RRS1B/RPS4B-dependent defence genes fold induction triggered by AvrRps4 ( Fig. 4 and Supplementary Fig. 8 ). We also could not observe greater gene induction in Ws-2 compared with the either single mutants. We infer that RRS1/RPS4 and RRS1B/RPS4B independently activate defence genes to a level adequate for resistance in response to AvrRps4. In the rps4-21/rps4b-1 double mutant fold induction of defence genes triggered by Pf Pf0-1 (AvrRps4) is not different to Pf Pf0-1 (AvrRps4 KRVY AAAA ), but is significantly lower than in AvrRps4-treated Ws-2 or single mutants ( Fig. 4 ). This means AvrRps4-triggered defence genes induction is fully dependent on functional RRS1B/RPS4B and/or RRS1/RPS4, which is consistent with the loss of resistance to Pst DC3000 (AvrRps4) observed in the double mutants ( Fig. 2d and Supplementary Fig. 1 ). Figure 4: Loss of RPS4 and RPS4B completely abolishes AvrRps4-triggered defence gene induction in Ws-2. Quantitative RT–PCR showing fold change of SARD1 , SID2 , EDS5 and PAD4 gene expression. Transcript levels were estimated in leaves of 5-week-old Ws-2, Ws-2 rps4-21 and rps4b-1 single and Ws-2 rps4-21 / rps4b-1 double mutants infiltrated with either H 2 O, Pf Pf0-1 secreting AvrRps4 KRVY AAAA or AvrRps4. RNA was extracted from samples taken at 6 h.p.i. for cDNA synthesis. Results of quantitative RT–PCR for selected defence marker genes were first normalized to EF1α , then calculated as log 2 -scaled fold change compared with H 2 O treatment. Means±s.e. of three biological replicates per sample are given. Data from individual experiments are shown in Supplementary Fig. 7 . Differences that are statistically significant are indicated (Student’s t -test * P≤ 0.05, ** P≤ 0.01, *** P≤ 0.001). Full size image RRS1B and RPS4B associate and function together We have established that there are two R gene pairs with ~60% identity that function independently to recognize AvrRps4 ( Supplementary Figs 9 and 10 ). Therefore, we wanted to understand how these R proteins work with their specific pair partners. Genetic evidence of pair specificity was shown in Fig. 2c where the RRS1B + RPS4 combination in Ws-2 rrs1-1/rps4b-1 cannot give HR to Pf Pf0-1 (AvrRps4). Similarly, the RRS1 + RPS4B combination in Col-0 rps4-2/rrs1b-1 does not give resistance to Pst DC3000 (AvrRps4; Fig. 2d ). In an N. tabacum transient assay, co-expression of RRS1-R + RPS4B or RRS1B + RPS4 combinations did not give HR to either AvrRps4 or PopP2 ( Fig. 5a,b and Supplementary Fig. 11 ). In contrast, popP2 only triggered HR when co-expressed with RRS1-R + RPS4 , and avrRps4 -triggered HR with both RRS1-R + RPS4 and RRS1B + RPS4B ( Fig. 5a ). This confirms that each R protein requires its cognate pair partner for function. 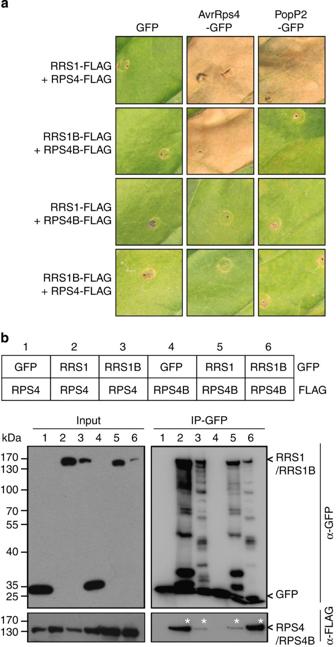Figure 5: Corresponding pair partner associationin plantais required for function. (a) HR assay inN. tabacumleaves using transientA. tumefacienstransformation. Each leaf section was co-infiltrated to express a different combination ofRgenes (shown on the left) together withGFP,avrRps4-GFPorpopP2-GFP.RRS1,RPS4,RRS1BandRPS4Bwere cloned from Ws-2 gDNA. Cell death pictures were taken 5 d.p.i. (b) Co-immunoprecipitation (co-IP) analysis showing associations within and between RRS1/RPS4 and RRS1B/RPS4B pair proteins.RRS1,RPS4,RRS1BandRPS4Bwere fused to either a C-terminal FLAG or GFP tag. The combination of fusion proteins in each sample (C-terminal tag indicated on the right) is listed in the panel with a corresponding number (1–6). Immunoblots show the presence of proteins in total extracts (Input) and after IP with anti-GFP beads (IP-GFP). Asterisks indicate the presence of protein bands after co-IP. These experiments were repeated at least three times with similar results. Figure 5: Corresponding pair partner association in planta is required for function. ( a ) HR assay in N. tabacum leaves using transient A. tumefaciens transformation. Each leaf section was co-infiltrated to express a different combination of R genes (shown on the left) together with GFP , avrRps4 - GFP or popP2 - GFP . RRS1 , RPS4 , RRS1B and RPS4B were cloned from Ws-2 gDNA. Cell death pictures were taken 5 d.p.i. ( b ) Co-immunoprecipitation (co-IP) analysis showing associations within and between RRS1/RPS4 and RRS1B/RPS4B pair proteins. RRS1 , RPS4 , RRS1B and RPS4B were fused to either a C-terminal FLAG or GFP tag. The combination of fusion proteins in each sample (C-terminal tag indicated on the right) is listed in the panel with a corresponding number (1–6). Immunoblots show the presence of proteins in total extracts (Input) and after IP with anti-GFP beads (IP-GFP). Asterisks indicate the presence of protein bands after co-IP. These experiments were repeated at least three times with similar results. Full size image RRS1 and RPS4 physically associate to form a functional recognition complex in planta [24] . Therefore, we tested by co-immunoprecipitation (co-IP) whether RRS1B and RPS4B also associate in planta , and if this association is specific to pair partners. Similar to RRS1-GFP and RPS4-FLAG, RRS1B-GFP co-IP with RPS4B-FLAG when transiently co-expressed in Nicotiana benthamiana leaves ( Fig. 5b lanes 2 and 6, and Supplementary Fig. 12 ). Interestingly, we also found RRS1B-GFP co-IP with RPS4-FLAG, and RRS1-GFP co-IP with RPS4B-FLAG ( Fig. 5b lanes 3 and 5 and Supplementary Fig. 12 ). However, the intensity of the co-IP signals was notably higher with the appropriate pair partners than with the inappropriate partners. We infer that the complexes formed of inappropriate pairing (for example, RRS1 + RPS4B or RRS1B + RPS4) are less stable, which could explain their non-functionality. Collectively, similar to RRS1/RPS4, RRS1B/RPS4B associate in planta to form a complex before any effector perception, and R protein pair complexes are only functional when formed of the appropriate partners. RRS1B and RPS4B TIR domains associate in planta TIR domains are considered to play a crucial role in defence activation as some of them can trigger immune responses when overexpressed alone in planta [32] , [33] , [34] , [35] , [36] . We showed overexpression of RPS4 TIR (1–235 a.a.)-triggered cell death in N. tabacum , whereas RRS1 TIR (1–175 a.a.) did not ( Fig. 6a ), consistent with previous report [24] . Interestingly, neither RPS4B TIR (1–235 a.a.) nor RRS1B TIR (1–166 a.a.) triggered cell death when overexpressed in N. tabacum ( Fig. 6a ). This implies either polymorphisms in RPS4B TIR compared with RPS4 TIR abolish its capacity to activate cell death or that N. tabacum lacks a components required for RPS4B TIR -triggered cell death. 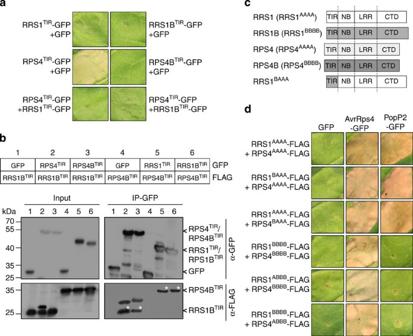Figure 6: The TIR domains of RRS1/RPS4 and RRS1B/RPS4B do not confer recognition or association specificity. (a) HR assay inN. tabacumleaves usingA. tumefaciens-mediated transient expression ofRRS1,RPS4,RRS1BandRPS4BTIR domains. Each leaf section was co-infiltrated by either single TIR domain with GFP control or by different TIR domain combinations. Cell death pictures were taken 5 d.p.i. (b) Co-IP analysis showing association of TIR domains from respective or different pair partners. TIR domains ofRRS1,RPS4,RRS1BandRPS4Bwere cloned from Ws-2 gDNA and fused to either a C-terminal FLAG or GFP tag. The combination of fusion proteins in each sample (C-terminal tag indicated on the right) is listed in the panel with a corresponding number (1–6). Immunoblots show the presence of proteins in total extracts (Input) and after IP with anti-GFP beads (IP-GFP). Asterisks indicate the presence of protein bands after co-IP. (c) Schematic representation of RRS1, RRS1B, RPS4, RPS4B from Ws-2, and a chimera protein RRS1BAAA. Each protein was shown with domain structure: RRS1 or RRS1B as TIR-NB-LRR-CTD (C-Terminal Domain)-WRKY; RPS4 or RPS4B as TIR-NB-LRR-CTD. Each domain is indicated with an ‘A’ or ‘B’, depending on which pair they belong to: RRS1/RPS4 (‘A’ pair), RRS1B/RPS4B (‘B’ pair). (d) HR assay inN. tabacumleaves using transientA. tumefacienstransformation. Each leaf section was co-infiltrated to express a different combination of WT and chimera proteins with TIR domains exchanged between ‘A’ pair and ‘B’ pair proteins (shown on the left) together withGFP,avrRps4-GFPorpopP2-GFP. RRS1BAAAand RRS1ABBBwere generated by swapping sequences coding for TIR domains between RRS1 and RRS1B. RPS4BAAAand RPS4ABBBwere generated similarly. Cell death pictures were taken 5 d.p.i. These experiments were repeated at least three times with similar results. Figure 6: The TIR domains of RRS1/RPS4 and RRS1B/RPS4B do not confer recognition or association specificity. ( a ) HR assay in N. tabacum leaves using A. tumefaciens -mediated transient expression of RRS1 , RPS4 , RRS1B and RPS4B TIR domains. Each leaf section was co-infiltrated by either single TIR domain with GFP control or by different TIR domain combinations. Cell death pictures were taken 5 d.p.i. ( b ) Co-IP analysis showing association of TIR domains from respective or different pair partners. TIR domains of RRS1 , RPS4 , RRS1B and RPS4B were cloned from Ws-2 gDNA and fused to either a C-terminal FLAG or GFP tag. The combination of fusion proteins in each sample (C-terminal tag indicated on the right) is listed in the panel with a corresponding number (1–6). Immunoblots show the presence of proteins in total extracts (Input) and after IP with anti-GFP beads (IP-GFP). Asterisks indicate the presence of protein bands after co-IP. ( c ) Schematic representation of RRS1, RRS1B, RPS4, RPS4B from Ws-2, and a chimera protein RRS1 BAAA . Each protein was shown with domain structure: RRS1 or RRS1B as TIR-NB-LRR-CTD (C-Terminal Domain)-WRKY; RPS4 or RPS4B as TIR-NB-LRR-CTD. Each domain is indicated with an ‘A’ or ‘B’, depending on which pair they belong to: RRS1/RPS4 (‘A’ pair), RRS1B/RPS4B (‘B’ pair). ( d ) HR assay in N. tabacum leaves using transient A. tumefaciens transformation. Each leaf section was co-infiltrated to express a different combination of WT and chimera proteins with TIR domains exchanged between ‘A’ pair and ‘B’ pair proteins (shown on the left) together with GFP , avrRps4 - GFP or popP2 - GFP . RRS1 BAAA and RRS1 ABBB were generated by swapping sequences coding for TIR domains between RRS1 and RRS1B. RPS4 BAAA and RPS4 ABBB were generated similarly. Cell death pictures were taken 5 d.p.i. These experiments were repeated at least three times with similar results. Full size image Many lines of evidence suggest TIR–TIR interactions are important for TNL function [24] , [37] . The TIR domains of RRS1 and RPS4 interact in a yeast two hybrid assay and associate in planta after co-IP [24] . TIR domains of these proteins are essential for effector recognition and defence activation [24] . In the pre-activation state, the RRS1/RPS4 heterodimer is proposed to be inactive. This correlates with the RRS1 TIR suppression of RPS4 TIR -triggered cell death when the TIR domains of these two paired R proteins associate ( Fig. 6a ) [24] . Interestingly, we found that RRS1B TIR can also suppress RPS4 TIR -triggered cell death ( Fig. 6a ), suggesting that TIR domains from different pairs can interact. Therefore, we investigated whether RRS1B TIR and RPS4B TIR can associate with each other in planta , and whether they can associate with RPS4 TIR and RRS1 TIR , respectively, by co-IP. After agro-infiltration in N. benthamiana , RRS1B TIR -FLAG co-IP with both RPS4B TIR -GFP and RPS4 TIR -GFP; and RPS4B TIR -FLAG co-IP with both RRS1B TIR -GFP and RRS1 TIR -GFP ( Fig. 6b and Supplementary Fig. 13 ). This suggests that, similar to full-length proteins, RRS1B TIR and RPS4B TIR can heterodimerize and also associate with RPS4 TIR and RRS1 TIR , respectively, in planta . TIR swaps between R protein pairs retain function We next assessed if, despite association of TIR domains between non-paired R proteins, the TIR domains contribute to the specificity of R protein function with each respective pair partner. To answer this question, we constructed chimeras in which RRS1 Ws-2 and RRS1B Ws-2 TIR domains were exchanged, and similarly with RPS4 Ws-2 and RPS4B Ws-2 TIR domains. We designated the four domains of RRS1 and RPS4 (TIR, NB, LRR and C-Terminal Domain) as ‘AAAA’ and of RRS1B and RPS4B as ‘BBBB’, defining TIR domain swaps as RRS1 BAAA and RRS1 ABBB full-length chimeric proteins ( Fig. 6c ). These chimeras were tested with WT R proteins for AvrRps4 and PopP2 recognition in N. tabacum transient assay. Similar to RRS1 AAAA and RPS4 AAAA , RRS1 BAAA +RPS4 AAAA and RRS1 AAAA +RPS4 BAAA combinations recognized both AvrRps4 and PopP2 ( Fig. 6d ). On the other hand, similar to RRS1 BBBB and RPS4 BBBB , RRS1 ABBB +RPS4 BBBB and RRS1 BBBB +RPS4 ABBB recognized AvrRps4 only ( Fig. 6d ). Accumulation of chimeric proteins was confirmed by immunoblot ( Supplementary Fig. 14a,b ). These results show that exchange of TIR domains from paralogous R genes does not compromise AvrRps4 or PopP2 recognition. In addition, the TIR domains do not drive the pair partner specificity for function, therefore other domain–domain interactions must account for the pairing specificity. We also characterized additional domain swaps between RRS1 and RRS1B, with the breakpoint between the end of exon 4 and the beginning of exon 5. Exons 5, 6 and 7 encode the WRKY domain of these proteins and ~260 amino acids between the LRR domain and the WRKY domain. These swaps were designated as ‘AAAB’ and ‘BBBA’, and tested for recognition of AvrRps4 and PopP2 in the presence of either RPS4 or RPS4B. Accumulation of chimeric proteins was confirmed by immunoblot ( Supplementary Fig. 14c, d ). Neither of the RRS1 AAAB and RRS1 BBBA chimeras conferred recognition of AvrRps4 or PopP2 ( Supplementary Fig. 15 ). However, RRS1 AAAB in combination with RPS4 showed constitutive activity and triggered cell death in the absence of effector, but not in combination with RPS4B ( Supplementary Fig. 15 ). This suggests that integrity and appropriate interactions in the C-terminal regions of these proteins might be required to prevent effector-independent defence activation. RRS1B associates with AvrRps4 and PopP2 in planta Recently, it was shown that the RRS1-R/RPS4 R protein complex associates with AvrRps4 and PopP2 in planta [24] . RRS1 and PopP2 were also shown to interact in a yeast split-ubiquitin assay [13] . However, this interaction is not sufficient for R protein activation as PopP2 also interacts with RRS1-S Col-5 but does not trigger an immune response in Col-5 (ref. 13 ). We examined whether RRS1B/RPS4B can also associate with AvrRps4 and also PopP2 in planta even if RRS1B/RPS4B cannot recognize PopP2. We co-expressed RRS1 Ws-2 -FLAG+RPS4 Ws-2 -FLAG and RRS1B Ws-2 -FLAG+RPS4B Ws-2 -FLAG , with either GFP , avrRps4-GFP or popP2-GFP in N. benthamiana . The GFP protein alone did not co-IP with the RRS1/RPS4 and RRS1B/RPS4B complexes ( Supplementary Figs 16 and 17 ). Similar to RRS1/RPS4 complex, RRS1B/RPS4B complex co-IP with both AvrRps4-GFP and PopP2-GFP ( Supplementary Figs 16 and 17 ). Interestingly, the signal intensity for RRS1/RPS4 was much stronger compared with RRS1B/RPS4B, indicating the RRS1/RPS4 complex has stronger affinity for both effectors than the RRS1B/RPS4B complex. Despite this observation, this result suggests that RRS1B/RPS4B associates in planta with AvrRps4 but also with PopP2. However, we cannot exclude that AvrRps4 and PopP2 break the pre-formed R protein heterodimer to associate with each of the partner separately. Considering the high intensity of RRS1 protein bands compared with RPS4 after AvrRps4 and PopP2 IP, we then tested whether RRS1 and RRS1B alone could associate with these effectors. Consistent with Williams et al . [24] , RRS1 co-IP with both AvrRps4 and PopP2 ( Fig. 7 lanes 3 and 5, and Supplementary Fig. 18 ) [24] . Interestingly, RRS1B also co-IP with both AvrRps4 and PopP2 ( Fig. 7 lanes 4 and 6, and Supplementary Fig. 18 ). Like in complex with their partner, RRS1 showed a stronger association with AvrRps4 and PopP2 than RRS1B. Altogether, this suggests that, similar to RRS1-S/RPS4 (ref. 13 ), protein–protein association of PopP2 with RRS1B/RPS4B can be detected but this is not sufficient for defence activation. 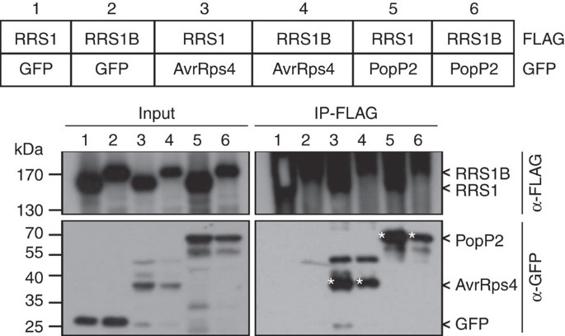Figure 7: Similar to RRS1, RRS1B associates with AvrRps4 and PopP2in planta. Co-IP analysis showing association of RRS1 and RRS1B with AvrRps4 and PopP2.RRS1andRRS1Bwere cloned from Ws-2 gDNA. The combination of fusion proteins in each sample (C-terminal tag indicated on the right) is listed in the panel with a corresponding number (1 to 6). Immunoblots show the presence of proteins in total extracts (Input) and after IP with anti-FLAG beads (IP-FLAG). Asterisks indicate the presence of protein bands after co-IP. Figure 7: Similar to RRS1, RRS1B associates with AvrRps4 and PopP2 in planta . Co-IP analysis showing association of RRS1 and RRS1B with AvrRps4 and PopP2. RRS1 and RRS1B were cloned from Ws-2 gDNA. The combination of fusion proteins in each sample (C-terminal tag indicated on the right) is listed in the panel with a corresponding number (1 to 6). Immunoblots show the presence of proteins in total extracts (Input) and after IP with anti-FLAG beads (IP-FLAG). Asterisks indicate the presence of protein bands after co-IP. Full size image Pair duplication and gain of WRKY domain in the Brassicaceae To shed some light on the evolution of these tandem paired R genes, we examined the genomes of several species related to A. thaliana , Using the nucleotide sequences of each gene from each pair in megablast searches [38] , we found that in the genomes of the sister species Arabidopsis lyrata [39] , and the closely related species Capsella rubella [40] , there are distinct putatively orthologous pairs matching both the ‘A’ pair ( RRS1/RPS4 ) and ‘B’ pair ( RRS1B/RPS4B ). In A. lyrata , we also found an apparent duplication of the ‘B’ pair, resulting in a paralogous ‘C’ pair with a high level of identity to the ‘B’ pair ( Fig. 8b,c ). Genome to genome comparison revealed that the regions of the A. thaliana , C. rubella and A. lyrata genomes harbouring the linked pairs were syntenic, with broad conservation of DNA sequence similarity and directionality ( Supplementary Fig. 19 ). Although highly syntenic, the region in A. lyrata is expanded in comparison to A. thaliana and C. rubella ( Supplementary Fig. 19 ). Additionally in A. lyrata , we found a divergently transcribed pair of TNL-encoding genes (gene names: 9301337 and 9301336) with similar identity to both the ‘A’ and ‘B’ pairs, which we named AlRPS4 -like and AlRRS1 -like, respectively ( Fig. 8a–c ). The RRS1- like gene of this pair, however, lacks the WRKY protein-encoding sequence, which is fused to RRS1 and RRS1B . Inspection of the DNA sequence directly following this RRS1- like gene confirmed that this was not due to the presence of an early stop codon. We also examined the genome of the more distant Arabidopsis relative Brassica rapa [41] . In the B. rapa genome, we found no WRKY-fused NB-LRR-encoding genes. A single B. rapa gene pair (gene names: Bra027598 and Bra027599 ) had the highest identity to the A. thaliana ‘A’ and ‘B’ pairs and is located in a region syntenic to the ‘A’ and ‘B’ region on A. thaliana chromosome 5 ( Fig. 8a–c and Supplementary Fig. 20 ). This pair lacks a WRKY fusion, and shows the highest nucleotide and protein level identity with AlRPS4 -like and AlRRS1 -like. We therefore speculate that these are the ancestors of the ‘A’, ‘B’ and ‘C’ pairs lacking the WRKY fusion. The B. rapa RRS1- like gene ( Bra027598 ) is fused to another, distantly related, TIR-NB-LRR-encoding gene at its 3′ end, although this may be a genome assembly or gene prediction artefact. Only the RRS1 -like half was used for the analyses presented. Although their amino-acid sequences have diverged, we found that the DNA sequences of each species’ RRS1 or RRS1B/C WRKY domain had the highest nucleotide identity and longest alignment to AtWRKY35 (selected alignments in Supplementary Fig. 21 ). These results suggest that a duplication of the ancestral pair fused with the sequence of a WRKY35- like gene in the common ancestor of A. thaliana , C. rubella and A. lyrata . Later in this common ancestor, a duplication event produced the ‘A’ and ‘B’ pairs. Specifically in the A. lyrata lineage, a further duplication of the ‘B’ pair occurred, resulting in the ‘C’ pair. 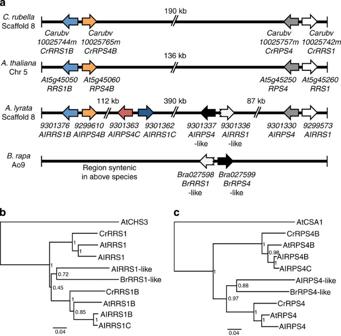Figure 8:RRS1/RPS4-likeRgene pair orthologues and progenitors in theBrassicaceae, (a) Schematic of theRRS1/RPS4-likeRgene pairs in variousBrassicaceaespecies. We identified the putative orthologues ofRRS1/RPS4andRRS1B/RPS4BinA. lyrataandC. rubella, HypotheticalRRS1-like genes that lack a WRKY domain are denoted with a broken tailed arrow inA. lyrataandB. rapa. Synteny was observed in theRRS1/RPS4region, although at varying scales (Supplementary Figs 14 and 15). TheAlRRS1C/AlRPS4Cpair is unique toA. lyrataand carries a WRKY domain (and is likely a more recent duplication of the B pair). The gene names noted refer to inC. rubellaandB. rapathe Phytozome database, inA. thalianathe TAIR database and inA. lyratathe NCBI RefSeq database. (b) RRS1 orthologues and paralogues cluster into distinct ‘A’, ‘B’ and ‘-like’ (non-WRKY) clades. Neighbour-joining tree based on the alignment of the amino-acid sequences of the various RRS1, RRS1-like proteins and a more distantly related outgroup, CHilling Sensitive 3 (CHS3)64. The numbers at nodes represent their bootstrap support (% support out of 1,000 bootstraps). The scale bar represents the number of amino-acid substitutions per site. (c) RPS4 orthologues and paralogues cluster into distinct ‘A’, ‘B’ and ‘-like’ clades. Neighbour-joining tree based on the alignment of the amino-acid sequences of the various RPS4- and RPS4-like proteins and a more distantly related outgroup, Constitutive Shade Avoidance 1 (CSA1)65. The numbers at nodes represent their bootstrap support (% support out of 1000 bootstraps). The scale bar represents the number of amino-acid substitutions per site. Figure 8: RRS1 / RPS4 -like R gene pair orthologues and progenitors in the Brassicaceae , ( a ) Schematic of the RRS1 / RPS4 -like R gene pairs in various Brassicaceae species. We identified the putative orthologues of RRS1/RPS4 and RRS1B/RPS4B in A. lyrata and C. rubella , Hypothetical RRS1- like genes that lack a WRKY domain are denoted with a broken tailed arrow in A. lyrata and B. rapa . Synteny was observed in the RRS1 / RPS4 region, although at varying scales ( Supplementary Figs 14 and 15 ). The AlRRS1C / AlRPS4C pair is unique to A. lyrata and carries a WRKY domain (and is likely a more recent duplication of the B pair). The gene names noted refer to in C. rubella and B. rapa the Phytozome database, in A. thaliana the TAIR database and in A. lyrata the NCBI RefSeq database. ( b ) RRS1 orthologues and paralogues cluster into distinct ‘A’, ‘B’ and ‘-like’ (non-WRKY) clades. Neighbour-joining tree based on the alignment of the amino-acid sequences of the various RRS1, RRS1-like proteins and a more distantly related outgroup, CHilling Sensitive 3 (CHS3) [64] . The numbers at nodes represent their bootstrap support (% support out of 1,000 bootstraps). The scale bar represents the number of amino-acid substitutions per site. ( c ) RPS4 orthologues and paralogues cluster into distinct ‘A’, ‘B’ and ‘-like’ clades. Neighbour-joining tree based on the alignment of the amino-acid sequences of the various RPS4- and RPS4-like proteins and a more distantly related outgroup, Constitutive Shade Avoidance 1 (CSA1) [65] . The numbers at nodes represent their bootstrap support (% support out of 1000 bootstraps). The scale bar represents the number of amino-acid substitutions per site. Full size image This study revealed that RRS1B / RPS4B , an R gene pair paralogous and closely linked to RRS1 / RPS4 , also recognizes AvrRps4, but not PopP2. In this system, multiple paired R proteins cooperate in a specific manner for the recognition of several effectors from unrelated plant pathogens ( Supplementary Fig. 22 ). The evolutionary advantage for the plant to carry two R gene pairs recognizing the same effector, AvrRps4, is unclear. Conceivably, RRS1B / RPS4B , which recognizes AvrRps4, duplicated to create RRS1-R / RPS4 , recognizing AvrRps4 and PopP2. Although our analyses of the genomes of various relatives of A. thaliana could not reveal which of the two pairs is ancestral, we did uncover the probable pre-WRKY fusion ancestor of both pairs, present in B. rapa and A. lyrata . We also found that distinct orthologous pairs are conserved in the A. lyrata and C. rubella genomes, suggesting that there is a selective advantage to maintaining both pairs. Indeed, in A. lyrata the ‘B’ pair has further duplicated to produce a closely related ‘C’ pair. We speculate that the duplication of such R gene pairs might reduce the effect of purifying selection and increase the potential for one of the pairs to evolve new or expanded effector recognition capacity [42] . In addition, developing two or more similar recognition systems might enable the plant to maximize protection of an important cellular complex generally targeted by pathogen effectors. However, accession RLD lost both RRS1/RPS4 and RRS1B/RPS4B functions. Conceivably, RLD evolved in an environment not exposed to pathogens recognized by RRS1 / RPS4 and/or RRS1B / RPS4B , and mutating these two R gene pairs could enhance fitness if there is a cost to resistance. Another hypothesis is that mutating these R gene pairs would have avoided a hybrid incompatibility [43] . Indeed, mutations in RRS1 can cause auto-activity of the RRS1/RPS4 complex leading to growth arrest [44] and this could also be the case for RRS1B/RPS4B. The appropriate partners of each of RRS1/RPS4 and RRS1B/RPS4B are required for effector-triggered immunity. These proteins form heteromeric complexes in a resting state before effector perception ( Supplementary Fig. 22a ). In addition, heteromeric complexes can be formed between partners from different pairs before effector recognition. However, such complexes are not functional for AvrRps4 and PopP2 recognition and/or downstream signalling activation. Altogether, this indicates that despite the similarity in motif prediction, TNLs evolved particular inter-molecular specificity for function. The TIR domains are not responsible for this phenomenon, and this specificity must be conferred by domains elsewhere in the R protein. However, we cannot exclude that association between WT proteins and TIR domains from different pairs is the result of overexpression in N. benthamiana , which might not occur under native expression. Integrity of NB-LRR protein is an important factor for function. Swapping parts of NB or LRR domains between the Rx and Gpa2 protein disrupt specific intra-molecular interactions and generate auto-active phenotype [45] , [46] . Similarly, we attempted to define the domains of RRS1-R responsible for PopP2 recognition by domain swaps with RRS1B. Although we did not identify this domain in this study, we were able to show that a combination of the RRS1 AAAB chimera with RPS4, but not with RPS4B, resulted in effector-independent HR. We infer that appropriate interactions between multiple domains in the complex are required to create a functional but not auto-active complex. Additional domain swap experiments between the two pairs will provide an opportunity for further mechanistic investigation. Several TNL s have been shown to recognize an effector directly and this direct interaction is presumed to trigger R protein activation [13] , [47] , [48] , [49] . The exact mechanism by which RRS1/RPS4 and RRS1B/RPS4B recognize AvrRps4 and PopP2 has not yet been reported. Although we only showed protein association by co-IP, we can speculate that the potential direct interaction of AvrRps4 with RRS1/RPS4 and RRS1B/RPS4B triggers R protein intra-molecular reconfigurations (and perhaps changes in oligomerization) leading to defence activation ( Supplementary Fig. 22b ). Such mechanisms could also be suggested for PopP2 recognition but, even if RRS1B/RPS4B associate with PopP2, this association does not trigger immunity. Therefore, an additional molecular event, occurring in the RRS1/RPS4/PopP2 but not in RRS1B/RPS4B/PopP2 complex, might be required ( Supplementary Fig. 22c ). Both RRS1 and RRS1B carry WRKY domains in their C-termini. WRKY domain-containing proteins play crucial roles in regulating plant defence [50] . If AvrRps4 and PopP2 virulence activities are to target WRKY domain-containing proteins, we could hypothesize that RRS1 and RRS1B, in association with RPS4 and RPS4B, respectively, could behave as decoys for effectors [44] , [51] . Intriguingly, at the nucleotide level, the WRKY domain of all the RRS1 orthologues and paralogues shows the highest identity to WRKY35 , suggesting a common origin. Despite this, the amino-acid sequence of the WRKY domain of RRS1B (WRKY16) is phylogenetically in group IIe of WRKY transcription factors, whereas that of RRS1 (WRKY52) lies in Group III (ref. 52 ). Conceivably, following duplication, differential adaptive changes occurred in the WRKY domains. If these domains are involved in effector recognition, the two R gene pairs may confer recognition of different subsets of WRKY-targeting effectors or effector alleles. Therefore, an important challenge is now to determine the precise role of each RRS1/RPS4 and RRS1B/RPS4B domain, and particularly to identify which of these domain(s) interact with AvrRps4 and PopP2. Also, identification of R protein complex components before and after effector recognition will help us to understand how TNL proteins function to activate plant immunity ( Supplementary Fig. 22d,e ). In summary, our data reveal an answer to a long-standing puzzle of how an Arabidopsis Col-0 or Ws-2 rps4 mutant can still activate defence in response to AvrRps4. We show that the RRS1B/RPS4B resembles structurally and functionally the RRS1/RPS4 pair. The RRS1/RPS4 and RRS1B/RPS4B gene pairs will be the subject of future investigations into the molecular and structural requirements that underpin how pair partner specificity occurs and how an interaction with AvrRps4 or PopP2 is converted into defence activation. Plant materials and growth conditions A. thaliana , N. benthamiana and N. tabacum (cultivar ‘Petit Gerard’) seeds were sown on compost and vernalized for 7 days (dark, 4 °C). Seedlings and adult plants were grown under controlled conditions: 21–23 °C; 10 h light/14 h dark; 75% humidity for Arabidopsis ; 21–23 °C; 16 h light/8 h dark; 55% humidity for Nicotiana sp . The Arabidopsis T-DNA insertion lines used in this study were obtained from the SALK and INRA institutes: At5g45050-1 ( 050-1 ) in Col-0 (SALK_001360), At5g45060-1 ( 060-1 ) in Ws-2 (FLAG_049F09); At5g45060-2 ( 060-2 ) in Col-0 (SALK_063382); rrs1-3 in Col-0 (SALK_061602); rps4-2 in Col-0 (SALK_057697). T-DNA insertions were confirmed by PCR using a specific primer of the T-DNA bordure (LBb1.3 primer for SALK lines: 5′-ATTTTGCCGATTTCGGAAC-3′; LB4 primer for FLAG lines: 5′-CGTGTGCCAGGTGCCCACGGAATAGT-3′) and a gene-specific primer ( Supplementary Table 2 ). Lack of expression of the knockout genes was confirmed by RT–PCR ( Supplementary Figs 2 and 3 and Supplementary Table 3 ). Stable transformation using floral dip method [53] was performed on 6- to 7-week-old flowering Arabidopsis plants. Genes of interest were amplified from gDNA with specific primers ( Supplementary Table 5 ), cloned into pENTR/D/TOPO and transferred into binary vector pBGW (using Gateway System) for Agrobacterium -mediated stable transgenic expression in planta . From dipped plants, T1 seeds were harvested, sterilized and selected either by spraying soil tray with phosphinothricin, or by growing on GM medium (4.3 g l −1 MS salts, 0.1 g l −1 myoinositol, 0.59 g l −1 MES, 8 g l −1 Bacto agar, 1 ml l −1 1,000 × GM vitamin stock, which contains 0.1% thiamine, 0.05% pyridoxine and 0.05% nicotinic acid; pH 5.7) containing appropriate antibiotics. Following similar procedure, T2 and T3 seeds were screened to obtain homozygous stable transgenic lines. Bacterial infections For HR assay, P. fluorescens ( Pf ) Pf0-1 freshly grown on selective lysogeny broth (LB) agar plates (engineered with type III secretion system) [22] , carrying pVSP61::avrRps4 KRVY AAAA , pVSP61::avrRps4, pEDV6::popP2 or pML123::hopA1 were harvested and resuspended in 10 mM MgCl 2 to OD 600 =0.2 for infiltration. Leaves of 5-week-old Arabidopsis plants were hand-infiltrated using 1 ml needless syringe and kept for 20–24 h for symptom (leaf tissue collapse) development. For in planta bacterial growth assay, Pst DC3000 carrying either pVSP61 (empty vector) or pVSP61::avrRps4 were grown on selective LB agar plates and harvested similar to Pf Pf0-1 strains. Bacterial suspension in 10 mM MgCl 2 were adjusted to OD 600 =0.001 for infiltration. Leaves of 5-week-old Arabidopsis plants were hand-infiltrated and harvested 3 d.p.i. for bacterial count. Infected leaf samples (1 cm 2 ) were ground in 10 mM MgCl 2 , serially diluted, spotted on selective LB agar plates and kept at 28 °C for 2 days before counting. Bacterial growing conditions and plasmid mobilization (triparental mating) were performed following published protocols [23] . Quantitative RT–PCR experiments Leaves of 5-week-old Arabidopsis were snap frozen at 6 h.p.i. with water, Pf Pf0-1 producing AvrRps4 KRVY AAAA or AvrRps4 for RNA extraction. Total RNAs were extracted using TRI reagent (Sigma), and purified using Qiagen RNeasy columns following the manufacturer’s instructions. Integrity of RNAs was assessed by electrophoresis. The complementary DNA was synthesized from 5 μg RNA using SuperScript II Reverse Transcriptase (Invitrogen), and subjected to real-time PCR SYBR Green JumpStart Taq ReadyMix (Sigma) in the CFX96 Thermal Cycler (Bio-Rad) using specific defence marker gene primers ( Supplementary Table 4 ). Each reaction (~50 ng cDNA per reaction) was performed in triplicates, and the average threshold cycle (Ct) was used to quantify relative gene expression. The relative expression values of defence marker genes were determined using the comparative Ct method (2 ΔCt ) with EF1α ( At5g60390 ) as a reference—normalization. After normalization, the fold change of defence gene induction was calculated on the log 2 scale compared with water (H 2 O) infiltrated samples in each genetic background. Statistical analysis was done using Student’s t -test. Transient genes expression in Nicotiana sp Agrobacterium tumefaciens strain AGL1 carrying various binary constructs were used for transient gene expression and subsequent protein accumulation in Nicotiana tabacum (Petit Gerard) or Nicotiana benthamiana , Full-length avrRps4 (1–221 aa) and popP2 (149–488 a.a.) were cloned and assembled (using pENTR and Gateway System) into binary vector pK7FWG2 (with 35S promoter and C-terminal GFP fusion tag; Supplementary Table 5 ). Fragments or full-length RRS1, RPS4, RRS1B and RPS4B were amplified from Ws-2 or RLD gDNA for Golden Gate assembly [54] into binary vector pICH86988 (with 35S promoter and C-terminal FLAG or GFP fusion tag; Supplementary Table 5 ). TIR domains of RRS1 (1–175 aa), RPS4 (1–235 aa), RRS1B (1–166 aa), RPS4B (1–235 a.a.) were amplified from Ws-2 and assembled similarly into pICH86988 . Chimera proteins of RRS1 and RRS1B, RPS4 and RPS4B were generated by swapping fragments coding for corresponding domains from either protein ( Fig. 6c ). To generate RPS4B (Δ3829)RLD , a nucleotide deletion was performed at 3,829 bp in RPS4B RLD using the QuickChange II XL Site-Directed mutagenesis kit (Agilent). Standard electroporation method was used for transformation of A. tumefaciens AGL1. Transformed A. tumefaciens were grown in liquid L-medium supplemented with appropriate antibiotics for 24–48 h. Cells were harvested by centrifugation and resuspended at OD 600 =0.4–0.5 in infiltration medium (10 mM MgCl 2 , 10 mM MES, pH 5.6). For co-expression, all bacterial suspensions carrying individual constructs were adjusted to OD 600 =0.4–0.5 in the final mix for infiltration. Five-week-old N. benthamiana leaves or N. tabacum leaf sections were infiltrated with 1 ml needleless syringe. The infiltrated N. benthamiana leaves were taken off at 2 d.p.i. for total protein extraction and co-IP. N. tabacum programmed cell death was photographed 5 d.p.i. Immunoblot analysis and co-IP experiments Details of immunoblot analysis and co-IP experiments following Agrobacterium -mediated transient protein accumulation in N. benthamiana leaves were described previously [23] . Protein samples were prepared from N. benthamiana leaves 48 h.p.i. with A. tumefaciens . One infiltrated leaf was harvested and ground in liquid nitrogen. Proteins were extracted from ground tissues in GTEN buffer (10% glycerol, 100 mM Tris-HCl, pH 7.5, 1 mM EDTA, 150 mM NaCl) supplemented with 5 mM dithiothreitol, 1% (vol/vol) plant protease inhibitor cocktail (Sigma) and 0.2% (vol/vol) Nonidet P-40. Lysates were centrifuged 15 min at 20,000 g at 4 °C and aliquots of filtered supernatants were used as input samples. Immunoprecipitations were conducted on 1.5 ml of filtered extract incubated for 2 h at 4 °C under gentle agitation in the presence of 20 μl anti-FLAG M2 affinity Gel (A2220 Sigma-Aldrich) or GFP-Trap_A (gtm-20 ChromoTek). Antibody-coupled agarose beads were collected and washed three times in GTEN buffer, resuspended in 3 × SDS-loading buffer and denatured at 96 °C for 10 min. Proteins were separated by SDS–PAGE and analysed by immunoblotting using anti-FLAG M2-Peroxidase (HRP) (A8592 Sigma) or anti-GFP(B-2) HRP (sc-9996 Santa Cruz Biotechnology). We used 1/10,000 dilution of 200 μg ml −1 anti-FLAG and anti-GFP antibodies in 5% non-fat milk. RRIR mapping To positionally clone the RRIR locus, a segregating population was generated by crossing Ws-2 rps4-21 with RLD. The Ws-2 rps4-21 × RLD F1 progeny showed HR to Pf Pf0-1 (AvrRps4), although variation in HR intensity was observed compared with the Ws-2 rps4-21 parent ( Fig. 1 ). This observation suggested a semi-dominance of the RRIR-conferring locus from Ws-2; this weak phenotype was designated ‘hr’ in contrast to the ‘HR’ of Ws-2 rps4-21 . The F2 progeny derived from F1 was then phenotyped (for the presence or absence of HR to Pf Pf0-1 (AvrRps4)) and genotyped to map the RRIR locus ( Fig. 2a and Supplementary Table 1 ). After infiltration of 48 F2 plants with Pf Pf0-1 (AvrRps4), an approximate 1:2:1 ratio (8 (HR):28 (hr):12 (no HR); χ 2 =2, P =0.572) was observed. This segregation suggested that the RRIR was associated with a single semi-dominant locus. To confirm the ratio observed in F2, we tested the HR phenotype segregation in 8 F3 plants derived from each of the 48 individual F2. By classifying the F3 families (F2:3) into those that showed HR, and those non-segregating for the absence of HR, a 3:1 ratio was observed (37 F2:3 with (HR): 11 F2:3 (no HR); χ 2 =0.111, P =0.945). This confirmed the presence of a single locus for the RRIR. To map the RRIR locus, we obtained and tested a total of 48 F2 individuals that did not segregate for the absence of Pf Pf0-1 (AvrRps4)-triggered HR in F3. As AvrRps4 recognition segregates 3:1 in a Ws-2 × RLD cross [11] , RRIR is likely to be conferred by a locus that is closely linked to RRS1 / RPS4 . Therefore, we focused the mapping on the lower arm of the chromosome 5 ( Fig. 2a ), around RPS4 , where all tested loci were homozygous for an RLD genotype in the 48 F2 individuals. Consistent with our hypothesis, markers SS007 (designed on RPS4 ) and SS017 mapped 2.1 cM (2 recombinants out of 48 F2 plants tested) from the RRIR locus confirming that RRIR and RPS4 loci were linked but distinct. The markers DFR.1 and N5-20408832 mapped, respectively, 5.7 cM (5 recombinants out of 44 F2 plants tested) and 14.1 cM (13 recombinants out of 46 F2 plants tested) from RRIR . The two recombinants (that is, two chromosomes heterozygous for Ws-2 genotype at the marker position) identified with SS017 were also recombinants at the N5-20408832 marker. Interestingly, no recombinants were similarly identified by DFR.1 and SS017 ( Fig. 2a ). Thus, we concluded that the RRIR locus resided between DFR.1 and SS017. In this region, only four TNL-encoding genes are predicted in Col-0 ( TAO1 , LAZ5 , At5g45050 and At5g45060 ; Fig. 2a ) [55] . We focused on TNL-encoding genes for RRIR as AvrRps4-dependent recognition in Ws-2 is EDS1 dependent [25] . The SS117 marker was designed onto At5g45060 , a TNL divergently transcribed from At5g45050 . SS117 co-segregated with the RRIR locus (0 recombinants out of 48 F2 plants tested; Fig. 2a ). TAO1 contributes to disease resistance against Pst DC3000 carrying AvrB in Arabidopsis [56] and LAZ5 is required for the lesion mimic mutant acd11 (ref. 57 ). At5g45050 and At5g45060 were hitherto uncharacterized. Interestingly, like RRS1 and RPS4 , At5g45050 and At5g45060 are divergently transcribed and in a head-to-head configuration. The RRS1 / RPS4 and At5g45050 / At5g45060 pairs share similar exon/intron architecture ( Fig. 2b ). At5g45050 and At5g45060 are the closest homologues of RRS1 and RPS4, respectively, within the predicted TNL proteins (with 58% and 64% of identity, respectively) [55] . Analysis of RRS1/RPS4- like pairs in Brassicaceae We used nucleotide–nucleotide BLAST 2.2.29+ [58] , specifically the megablast algorithm [38] , to search the predicted coding sequence databases from A. lyrata [39] , C. rubella [40] and B. rapa [41] with the A. thaliana Col-0-coding sequences of RRS1, RPS4, RRS1B and RPS4B . Following the identification of putatively orthologous genes, MUSCLE [59] and CLUSTAL W [60] nucleotide and protein sequence alignments were used to generate phylogenetic trees using the Neighbour-Joining and Maximum Likelihood (Tamura-Nei model) methods, each with 1,000 bootstraps. These analyses were carried out within the MEGA 6 suite [61] . Note that the trees presented in Fig. 8 were constructed with CLUSTALW protein alignments and the Neighbour-Joining method and were consistent with the trees generated using the other methods. FigTree v1.4 ( http://tree.bio.ed.ac.uk/software/figtree/ ) was used to prepare the trees for publication. To determine the closest WRKY domain nucleotide sequence to the various RRS1 WRKY domain sequences, a database of all WRKY family genes in A. thaliana was searched using nucleotide–nucleotide megablast. Alignment of the nucleotide sequences of AtWRKY35 and RRS1 and RRS1B was accomplished using the EMBOSS MATCHER online tool [62] . To establish genome–genome synteny, the nucleotide sequences of the genomic regions harbouring the genes of interest were extracted and queried against each other using megablast. The tabular (output format 6) results were then loaded into the Artemis Genome Comparison Tool [63] , which was used to visualize and check for synteny across the various Brassicaceae RRS1/RPS4- encoding regions. How to cite this article: Saucet, S. B. et al . Two linked pairs of Arabidopsis TNL resistance genes independently confer recognition of bacterial effector AvrRps4. Nat. Commun , 6:6338 doi: 10.1038/ncomms7338 (2015).